Encapsulation kinetics and dynamics of carbon monoxide in clathrate hydrate Carbon monoxide clathrate hydrate is a potentially important constituent in the solar system. In contrast to the well-established relation between the size of gaseous molecule and hydrate structure, previous work showed that carbon monoxide molecules preferentially form structure-I rather than structure-II gas hydrate. Resolving this discrepancy is fundamentally important to understanding clathrate formation, structure stabilization and the role the dipole moment/molecular polarizability plays in these processes. Here we report the synthesis of structure-II carbon monoxide hydrate under moderate high-pressure/low-temperature conditions. We demonstrate that the relative stability between structure-I and structure-II hydrates is primarily determined by kinetically controlled cage filling and associated binding energies. Within hexakaidecahedral cage, molecular dynamic simulations of density distributions reveal eight low-energy wells forming a cubic geometry in favour of the occupancy of carbon monoxide molecules, suggesting that the carbon monoxide–water and carbon monoxide–carbon monoxide interactions with adjacent cages provide a significant source of stability for the structure-II clathrate framework. Clathrate hydrates are non-stoichiometric compounds consisting of various types of hydrogen-bonded water polyhedral cages containing guest molecules [1] . Depending on the cage geometry and connectivity, hydrates usually crystallize in one of the two most common structures, structure-I (sI, space group ) and structure-II (sII, ), both of which are cubic. The sI unit cell contains two pentagonal dodecahedra (5 12 ) cages and six tetradecahedron (5 12 6 2 ) cages. In a sII unit cell, there are 16 5 12 cages and 8 large hexakaidecahedral 5 12 6 4 cages. The structure formed largely depends on the size of guest molecules enclosed in the cages. sI is often formed with small guest molecules such as methane and carbon dioxide, while sII can enclose larger guests such as propane and isobutene. Interestingly, very small molecules, such as H 2 , N 2 and O 2 , also form sII hydrates. These molecules can stabilize the ice-like framework because sII has a larger number of small cages and because the large 5 12 6 4 cages can accommodate multiple small molecules. There is yet a third hydrate structure, known as structure H (sH) [1] , [2] , which crystallizes in a P 6/ mmm structure consisting of layers of 5 12 cages alternating with those of 4 3 5 6 6 3 and 5 12 6 8 cages. The 5 12 and 4 3 5 6 6 3 cages are occupied by small molecules such as methane while the molecules in the large interstitial icosahedral (5 12 6 8 ) cages are typically larger than 7 Å, such as neohexane and adamantane [1] , [3] . Therefore, the stabilization of the sH structure requires the enclosure of both small and large guest molecules. Generally speaking, multiple hydrate structures of small single gases such as CO 2 , N 2 , Xe, Kr and CH 4 (refs 4 , 5 , 6 , 7 , 8 , 9 , 10 ) can be formed at various pressure and temperature conditions. As a cosmochemically important gas molecule and a predominant form of carbon in solar nebulae [11] , carbon monoxide (CO) occurs in mixed gas hydrates (CO 2 , H 2 , N 2 and so on), and the formation of these clathrate phases may play important roles in the formation of nebulae, comets and the outer planets of the solar system [12] , [13] . For instance, the high CO/N 2 ratios in primordial Titan may indicate that CO had a higher possibility to form clathrate relative to N 2 if both gases were accreted as clathrates [12] . In addition, these enclosure compounds are environmentally relevant, as they have potential applications in the sequestration of greenhouse gases and separation of industrial flue gases. For a given method of measurement, a molecule of CO has a similar size to those of N 2 and O 2 ; consideration of only the size effect therefore favours a sII clathrate, based on the guest–hydrate cavity size relation [14] . In addition, based on the theoretical calculation, Miller [13] predicted that sII CO clathrate is energetically more favourable than its sI counterpart. However, contrary to this prediction, all experimental studies show that CO forms sI clathrate hydrate under moderate pressure and temperature conditions [15] , [16] , [17] , [18] , [19] , [20] . Thermodynamic calculations using the classical Lennard–Jones–Devonshire cell model also concluded that CO sI hydrate would be more stable, giving a dissociation pressure that is 20% lower than that for sII clathrate [12] . Recently, Dartois [20] modelled the equilibrium phase diagram of CO clathrate in P – T space using the Ballard and Sloan’s formalism [21] and the Kihara potential for CO [17] . The calculated stability curve for sII lies slightly below that for sI, indicating that the sII clathrate is thermodynamically favoured. To date, the controversy between experiments and theoretical predictions has not been resolved. One school of thought attributes the discrepancy to the electrostatic properties (that is, dipole moment and molecular polarizability) of the CO molecule during clathration. This hypothesis is worth exploring because the dipole moment is an important factor that influences the hydrate stability; other factors include the size of guest molecules, short range guest–host interactions and hydrogen bonding [22] . Unlike other molecules such as H 2 , CO 2 , CH 4 and especially N 2 , which is isoelectronic with CO, the CO molecule has a non-zero dipole moment of 0.122 D. The exact nature of the dipole interaction between CO and clathrate cages is not currently known. It has also been argued that the crystallization of CO clathrate requires high concentration of gaseous molecules to overcome a significant energy barrier to nucleation. As a result, nucleation would be more efficient in a pressure region where the sI CO clathrate is favoured [20] . In the absence of thermodynamic equilibrium data for the sII CO clathrate, such as framework stability and cage occupancy, one is left with an inconclusive hypothesis that warrants further experimental validation. In this work, we conduct time-dependent neutron diffraction experiments on the D 2 O(s)–CO(g) system at simultaneously low temperature and high hydrostatic pressure conditions. We successfully synthesize sII CO hydrate and determine its cage gas filling as a function of time. We also perform density functional theory (DFT) calculations to evaluate the thermodynamic properties of this system. On the basis of the obtained results, the stability of CO hydrates appears to be primarily controlled by the cage occupancy and the binding energy between CO and D 2 O molecules. Using combined analyses of Rietveld refinement, maximum entropy method (MEM) and molecular dynamics (MD) simulations, we investigate the distribution of CO molecules in sII cages and their interaction with, and stabilization in, the host water framework. 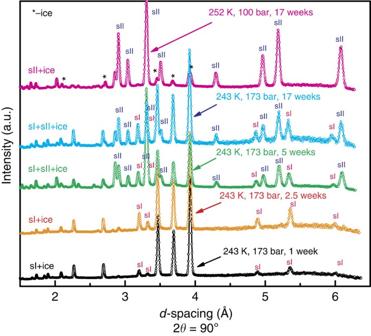Figure 1: Neutron diffraction data. Time-dependent neutron diffraction patterns showing carbon monoxide clathrate formation. The diffraction patterns collected at 173 bar after 1, 2.5 and 17 weeks are from one synthesis run. The patterns collected at 173 bar after 5 weeks and at 100 bar after 17 weeks are from another synthesis run. The conditions shown in the figure are the synthesis pressures and temperatures. All neutron diffraction data were obtained at 260 K and at indicated pressures. Neutron diffraction Figure 1 shows neutron diffraction patterns of CO hydrates obtained in two different synthesis experiments. Consistent with the earlier finding [15] , [16] , CO hydrate crystallized in sI at 173 bar and 243 K. Over the initial period of two and a half weeks, the CO gas continued to react with D 2 O ice to form sI hydrate. Interestingly, in both experiments, sII hydrate started to form and coexisted with sI hydrate after staying at the same conditions for additional amounts of time. These observations indicate that the formation of sII CO hydrate at these P – T conditions is thermodynamically favoured but not kinetically favoured. They also indicate that between the two competing pathways leading to CO hydrates, the activation energy for sI is lower than that for sII. Hence, the earlier nucleation of sI hydrate is kinetically controlled. Further inspection of Fig. 1 reveals that after the appearance of sII hydrate the relative diffraction intensities between sI and sII hydrates do not show notable changes with time, indicating that the two hydrates may have formed via two separate nucleation paths. When the pressure was decreased from 173 to 100 bar while the temperature was kept at 252 K for 12 weeks, a pure phase sII hydrate was finally obtained. To gain further insight into the kinetics of sII hydrate formation, we performed a third experiment at a lower pressure, 100 bar, and 252 K. However, neither sI nor sII hydrate was observed over a period of three and a half weeks. This is not totally unexpected because the formation of both sI and sII CO hydrates requires a threshold pressure to trigger the nucleation of the clathrate phase. Clearly, in the system CO(g)–D 2 O(s), the applied pressure of 100 bars was too low to fulfil this requirement. Figure 1: Neutron diffraction data. Time-dependent neutron diffraction patterns showing carbon monoxide clathrate formation. The diffraction patterns collected at 173 bar after 1, 2.5 and 17 weeks are from one synthesis run. The patterns collected at 173 bar after 5 weeks and at 100 bar after 17 weeks are from another synthesis run. The conditions shown in the figure are the synthesis pressures and temperatures. All neutron diffraction data were obtained at 260 K and at indicated pressures. Full size image In a given system, pressure and temperature are the most important thermodynamic parameters. From this point of view, it is quite unexpected that D 2 O ice first reacts with CO molecules to form sI hydrate at 173 bar and 243 K and then to form sII hydrate at the same P – T conditions, either through the same reaction or a phase transformation. However, composition is yet another important thermodynamic variable, especially for clathrate hydrates. Because hydrates are intrinsically non-stoichiometric, their compositions are closely tied to the filling of the cages, which would in turn influence their thermodynamic stability. To gain insight into this effect, we refined the cage occupancies using the data shown in Fig. 1 . Our results indicate that the small cages in sI and sII clathrates are fully or close to fully occupied (100±5% uncertainty); therefore, to a first approximation, they were fixed at a full occupancy during the subsequent refinements. For 5 12 6 2 cages in sI, the occupancies are 1.13, 1.18, 1.34 and 1.39, in hydrates synthesized for 1, 2.5, 5 and 17 weeks, respectively. For 5 12 6 4 cages in sII, they are 1.59 and 2, in hydrates synthesized for 5 and 17 weeks, respectively. As expected, the cage occupancies increase gradually on increasing the synthesis time. Note that, over a given period of time, the number of CO molecules in each 5 12 6 2 cage is substantially smaller than that in 5 12 6 4 cage. Theoretical calculation To understand the effects of cage occupancy on the stability of CO hydrates, we performed DFT calculations to determine the binding energies, Δ E , of CO m -(H 2 O) n clusters, which are calculated as where m and n are the numbers of enclosed CO and water molecules in the cage, respectively. The values of n corresponding to 5 12 , 5 12 6 2 and 5 12 6 4 cages are, respectively, 20, 24 and 28. Our optimized geometries for H 2 O cages are in good agreement with previous predictions by Patchkovskii et al. [23] For the CO-(H 2 O) 20 cluster, the calculated binding energies are 3.47 and 2.59 kcal mol −1 without and with zero point energy (ZPE) corrections, respectively. These values are comparable to the binding energy of the CO-H 2 O complex [24] . The optimized structure shows that a CO molecule occupies the centre of each 5 12 cage, with the C atom being 0.5 Å from the cage centre. This is consistent with the MD simulation results using a classical force field, which will be discussed later. Instead of forming a single CO-H 2 O complex, each CO molecule interacts with all surrounding H 2 O molecules. The binding energies without and with ZPE correction for CO-(H 2 O) 24 (5 12 6 2 cage) are 3.08 and 2.37 kcal mol −1 , respectively, and those for CO-(H 2 O) 28 (5 12 6 4 cage) are 2.76 and 2.14 kcal mol −1 , respectively. Thus, water molecules in larger cages tend to have weaker binding (specifically van der Waals interaction) with CO molecules due to their larger separation. For the two CO molecules encapsulated in either a 5 12 6 2 (sI) or 5 12 6 4 (sII) cage, several trial positions, such as cage centre and cage edges facing the hexagonal and pentagonal rings, were also explored for possible CO occupancies. In both cases, no breakdown in cage symmetries was found, and the CO molecules eventually became equilibrated at the stabilized positions. However, the calculated binding energies for the optimized (CO) 2 -(H 2 O) 28 cluster without and with ZPE are 2.68 and 1.12 kcal mol −1 , respectively, both of which are substantially lower than the sums of the corresponding binding energies for the two CO-(H 2 O) 28 clusters. The binding energies of (CO) 2 -(H 2 O) 24 cluster with the ZPE correction are found to be very low or even negative, which is obviously due to the size effect of the sI large cage (5 12 6 2 ). The occupation of two CO molecules in each 5 12 6 2 cage can therefore significantly destabilize the sI CO clathrate structure. 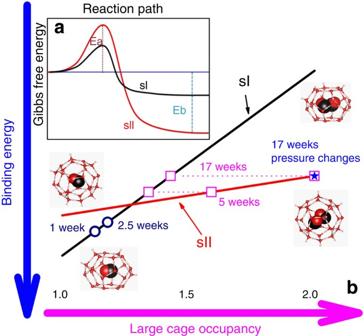Figure 2: Formation energetics of clathrate hydrates. (a) A schematic view of Gibbs free energy as a function of reaction coordinate for the formation of sI and sII carbon monoxide hydrates, inferred from our experimental observations (Fig. 1) and binding energy calculations. The horizontal line denotes the ground state of Gibbs free energy.EaandEbare activation energy and binding energy, respectively. The Gibbs free energy associated withEbis negative as binding energy is released; (b) a schematic illustration of cage occupancy in 51262and 51264cages as a function of binding energy in sI and sII carbon monoxide clathrates at pressure–temperature conditions near the phase boundary. Figure 2 shows a schematic plot of the calculated binding energies for single and double occupancies of CO molecules in the large cages of sI and sII clathrates. Strikingly, there is a crossover in binding energy, indicating that beyond a critical point of cage occupancy the 5 12 6 4 cages are energetically favoured over the 5 12 6 2 cages in the clathrate structure. Also plotted in Fig. 2 are the cage occupancies determined from the neutron data shown in Fig. 1 . The sI clathrate was initially observed after the synthesis time of 1 and 2.5 weeks because the 5 12 6 2 cages are energetically favoured at small cage occupancies. However, when CO molecules are concentrated over a long period of time, the energetics is in favour of the 5 12 6 4 cages enclosing two CO molecules and hence the sII hydrate. Our experiments show that relative to the sI phase, sII hydrate is thermodynamically favoured (lower Gibbs free energy) but not kinetically favoured (higher activation energy for the formation of stable, critical-sized hydrate nuclei). Therefore, at the final equilibrium state, sII hydrate must have higher binding energy than sI hydrate as illustrated in the inset of Fig. 2 . This thermodynamic view is qualitatively consistent with our binding energy calculations. As also shown in Fig. 2 , there is a region where sI and sII hydrates can coexist (marked by horizontal dot lines that intersect the two bold lines), which corresponds to the hydrates synthesized at 173 bar for 5 and 17 weeks. It should be pointed out that such coexistence can only be possible when P – T conditions are in the vicinity of the sI–sII hydrate phase boundary. As shown in the top pattern of Fig. 1 , a phase-pure sII CO clathrate was obtained when the synthesis pressure was significantly lowered. On the other hand, an increase in pressure at a given temperature would favour the formation of sI hydrate [20] . Figure 2: Formation energetics of clathrate hydrates. ( a ) A schematic view of Gibbs free energy as a function of reaction coordinate for the formation of sI and sII carbon monoxide hydrates, inferred from our experimental observations ( Fig. 1 ) and binding energy calculations. The horizontal line denotes the ground state of Gibbs free energy. E a and E b are activation energy and binding energy, respectively. The Gibbs free energy associated with E b is negative as binding energy is released; ( b ) a schematic illustration of cage occupancy in 5 12 6 2 and 5 12 6 4 cages as a function of binding energy in sI and sII carbon monoxide clathrates at pressure–temperature conditions near the phase boundary. Full size image Our calculated binding energies for the optimized (CO) 2 -(H 2 O) 28 clusters are substantially lower than the sum of the binding energies for two individual CO-(H 2 O) 28 clusters. Therefore, the (CO) 2 -(H 2 O) 28 clusters in an isolated state are energetically unfavourable and may readily dissociate into CO-(H 2 O) 28 +CO. However, the interaction between (CO) 2 -(H 2 O) 28 clusters and their adjacent cages may play an important role in stabilizing the doubly occupied 5 12 6 4 cages. The 5 12 6 4 cages in sII clathrate, for example, are tightly connected to other 5 12 cages and 5 12 6 4 cages by sharing pentagonal faces and hexagonal faces. To gain insight into the distribution of CO molecules in hydrate cages and their intra- and inter-cage interactions, we performed a combined analysis of Rietveld refinement, MEM and MD simulations. In sII CO hydrate, the 5 12 cages share pentagons to form linear chains along the [110] direction, and each 5 12 6 4 cage shares four hexagons with four neighbouring 5 12 6 4 cages to form a diamond-shaped cage centre ( Supplementary Fig. 1 ). The volume thermal expansion data were fitted to yield the parameters β =8.2(17) × 10 −6 K −1 and γ =8.7(2) × 10 −7 K −2 ( Supplementary Fig. 2 ). Because CO molecule is smaller than the cage size of 5 12 or 5 12 6 4 and because the interaction between CO and the cages is via weak van der Waals force and even weaker dipole interactions, CO molecules in both cages have a disordered distribution. 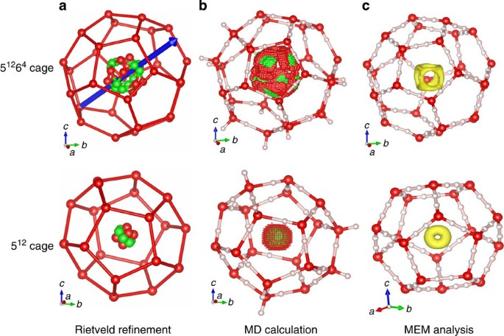Figure 3: Carbon monoxide distributions. The distribution of carbon monoxide molecules in 51264and 512cages at 25 K (a) from Rietveld refinement; (b) from MD simulations with the 10% top possibilities of carbon monoxide molecular trajectories (oxygen in red and carbon in green) (Supplementary Fig. 3); and (c) from MEM analysis with isosurface level of 1.5 fm Å−3for 51264cage and 3 fm Å−3for 512cage. The Pauling’s half-hydrogen model with an average occupancy of 0.5 for each deuterium atom in water molecules was used for the Rietveld refinement and MEM analysis, and the ordered model was used for MD calculation. The green balls represent possible positions of carbon atoms, and the red balls represent oxygen atoms. In a 51264cage, the 12-fold coordinated carbon and oxygen positions are each related by a three-fold symmetry axis, and are normal to the hexagonal faces along the body diagonal of the cubic unit cell. The carbon atoms point towards the four hexagons and oxygen atoms point towards the four co-vertexes of the three pentagons. In a 512cage, the sixfold coordinated carbon and oxygen positions are each related by a three-fold body-diagonal axis, and the distribution of the carbon–oxygen bonds forms a solid angle of 102.6°. The carbon positions form a donut-shape ring in between the oxygen positions. Figure 3 shows the distribution of CO molecules in 5 12 6 4 and 5 12 cages at 25 K. CO molecules partially occupy small and large cages with the occupancy of 1/6 ( Table 1 ). Difference Fourier nuclear maps reveal that CO molecules are off-centred, as also demonstrated by the CO distribution from MD simulations in Fig. 3b and nuclear density distribution from MEM in Fig. 3c . The off-centred character agrees well with the computed positions of the CO molecules in sI clathrate [18] , [25] . Note that, as a result of the disordered nature of guest molecules in the cages [22] , [26] , the described CO distribution is only one of the most probable structural configurations from our Rietveld analyses, which, however, does not provide insight into the dynamics of guest molecules in the cages. On the other hand, a previous nuclear magnetic resonance (NMR) study on sI clathrate shows [15] , [16] that the CO molecules in the large cages undergo anisotropic reorientation with substantial mobility even at 77 K. The proposed model involves rapid motion of CO molecules among sites over each of the 14 faces, with the CO axis orientated towards the cage centre. Clearly, other techniques, such as NMR, Raman, infrared and inelastic scattering spectroscopies, are needed to provide more comprehensive understanding of the disordered state and dynamics of CO molecules in sII clathrate cages. Figure 3: Carbon monoxide distributions. The distribution of carbon monoxide molecules in 5 12 6 4 and 5 12 cages at 25 K ( a ) from Rietveld refinement; ( b ) from MD simulations with the 10% top possibilities of carbon monoxide molecular trajectories (oxygen in red and carbon in green) ( Supplementary Fig. 3 ); and ( c ) from MEM analysis with isosurface level of 1.5 fm Å −3 for 5 12 6 4 cage and 3 fm Å −3 for 5 12 cage. The Pauling’s half-hydrogen model with an average occupancy of 0.5 for each deuterium atom in water molecules was used for the Rietveld refinement and MEM analysis, and the ordered model was used for MD calculation. The green balls represent possible positions of carbon atoms, and the red balls represent oxygen atoms. In a 5 12 6 4 cage, the 12-fold coordinated carbon and oxygen positions are each related by a three-fold symmetry axis, and are normal to the hexagonal faces along the body diagonal of the cubic unit cell. The carbon atoms point towards the four hexagons and oxygen atoms point towards the four co-vertexes of the three pentagons. In a 5 12 cage, the sixfold coordinated carbon and oxygen positions are each related by a three-fold body-diagonal axis, and the distribution of the carbon–oxygen bonds forms a solid angle of 102.6°. The carbon positions form a donut-shape ring in between the oxygen positions. Full size image Table 1 Refined structural parameters of carbon monoxide sII clathrate at 25 K. Full size table In the 5 12 6 4 cages of sII clathrate, there are eight low-energy wells in two different groups favouring the occupancy of CO molecules: four in one group facing the four hexagonal rings of the 5 12 6 4 cage, along the body diagonal of the unit cell, and the remaining four in the second group facing the co-vertex of three pentagonal rings of the 5 12 6 4 cage, also along the body diagonal. Together, these eight positions form a cubic geometry with an edge length of ~3 Å, which has the same orientation as the unit cell. In the 5 12 6 4 cages, CO molecules are distributed at the eight vertices of the cube, which is different from the oblate shape of the CO distribution at the 14 sites towards each face of 5 12 6 2 cage in sI clathrate [15] , [16] . Such distributions suggest that the intra-cage CO-H 2 O interaction and inter-cage CO-CO interaction can provide a significant source of stability for the sII framework. To corroborate this assumption, we have estimated the relative contribution of long-range interaction to the total stabilization of CO molecules in the large cage by calculating the trajectory average interaction energy of CO molecules within the 5 12 6 4 cage. The stabilization energy of a CO molecule provided by the 5 12 6 4 cage is determined to be ~65% of the total interaction energy of the CO molecule, indicating that the molecules in the adjacent cages contribute 35% of the interaction energy for CO molecules in the doubly occupied cages. We have also found that the interaction between CO molecules inside a single cage has negative contribution to the stabilization of the system by energy decomposition analysis. Both of these findings are in good agreement with the results of our DFT calculations. It is worth pointing out that the structure and thermodynamic stability of clathrate hydrates are generally determined by two main factors: intermolecular interaction between guest and host molecules and the configurational entropy. The present work has focused on the former, but the latter contribution to the Gibbs free energy can also be important for guest molecules that strongly interact with the host framework water molecules. In addition, the stabilization mechanism by the adjacent cage interaction is yet to be fully understood, which represents another important area for future investigations. In 5 12 cage, our MEM analysis demonstrates that CO molecules exhibit a doughnut-shaped density distribution, which is normal to the <111> cubic diagonals ( Fig. 3c ). Compared with the single occupancy in a 5 12 cage, the enclosure of two CO molecules in a 5 12 6 4 cage will increase the positional disorder and the scattering distributions (lower-symmetric position), which would in turn result in larger isotropic thermal motion ( U iso ) and displacement of CO from the cage centre. 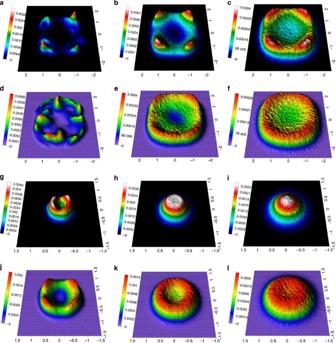Figure 4: Two-dimensional carbon monoxide distributions. The distribution of carbon monoxide molecules in sII clathrate from MD simulation: (a–c) carbon atoms in carbon monoxide in 51264cages at 25, 100 and 260 K, respectively; (d–f) oxygen atoms in carbon monoxide in 51264cages at 25, 100 and 260 K, respectively; (g–i) carbon atoms in carbon monoxide in 512cages at 25, 100 and 260 K, respectively; (j–l) oxygen atoms in carbon monoxide in 512cages at 25, 100 and 260 K, respectively; the intensities are projected on thea–bplane from around 10,000 carbon monoxide molecules. The cage centre is at coordinate (0,0), and the axial unit is Å. The intensity is the normalized density distribution of carbon monoxide in clathrate cages, and the summed total value is 1 in each cage. Figure 4 shows the detailed CO distributions in sII cages obtained from MD simulation. As is shown, both C and O atoms in CO molecules are distributed off the centre of the 5 12 6 4 cage. The a – b plane projection of the density distributions displays four overlapped intensity maxima for the CO positions in the 5 12 6 4 cage, indicating that the C atoms are localized with the O atoms rotating around them, even though the CO molecules are allowed to move freely in the 5 12 6 4 cage. Since such a configuration results from the combined effect of inter-cage CO-CO and CO-H 2 O interactions, the hollow shape of the CO distribution is expected to constitute a core that stabilizes both the 5 12 6 4 cage of sII clathrate and the CO dimer contained within. Increasing the temperature would further delocalize the distribution of CO molecules in the cages, but they would still be confined within the potential energy surface well ( Supplementary Fig. 4 ). Figure 4: Two-dimensional carbon monoxide distributions. The distribution of carbon monoxide molecules in sII clathrate from MD simulation: ( a – c ) carbon atoms in carbon monoxide in 5 12 6 4 cages at 25, 100 and 260 K, respectively; ( d – f ) oxygen atoms in carbon monoxide in 5 12 6 4 cages at 25, 100 and 260 K, respectively; ( g – i ) carbon atoms in carbon monoxide in 5 12 cages at 25, 100 and 260 K, respectively; ( j – l ) oxygen atoms in carbon monoxide in 5 12 cages at 25, 100 and 260 K, respectively; the intensities are projected on the a – b plane from around 10,000 carbon monoxide molecules. The cage centre is at coordinate (0,0), and the axial unit is Å. The intensity is the normalized density distribution of carbon monoxide in clathrate cages, and the summed total value is 1 in each cage. Full size image The radial distribution functions (RDFs) of CO molecules in sII clathrate from MD calculations are shown in Fig. 5 . For the 5 12 cage, the RDF is in excellent agreement with that reported for sI clathrate [18] , [24] . This is not unexpected given the similar cage geometries in sI and sII clathrates, even though the cages in the two structures have different symmetries. However, the RDF for CO molecules in the 5 12 6 4 cage is significantly different from that in sI [18] . The peak values of both C and O atoms are lower for sII than for sI. There is no zero point at any distance as in the case of sI. This suggests that in the large cage of sII hydrate, CO molecules are more delocalized than those in sI and hence have a smoother potential energy surface. Thus, the larger cage size in sII not only increases the binding energy but also significantly lowers the potential barriers for CO molecules to move. The delocalization behaviour of CO is similar to that of D 2 observed in hydrogen clathrate hydrate [27] , which also has a sII structure containing large 5 12 6 4 cages. Thus, like all other hydrates of small guest molecules, the guest–framework interactions in CO clathrate hydrates may be dominated by the delocalization of encapsulated molecules inside their cages. 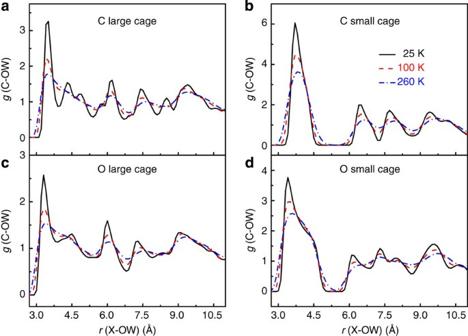Figure 5: Radial distribution function. Radial distribution functions of carbon atoms in carbon monoxide molecules in 51264(a) and 512(b) cages, and oxygen atoms in carbon monoxide molecules in 51264(c) and 512(d) cages at 25, 100 and 260 K from MD simulation. Figure 5: Radial distribution function. Radial distribution functions of carbon atoms in carbon monoxide molecules in 5 12 6 4 ( a ) and 5 12 ( b ) cages, and oxygen atoms in carbon monoxide molecules in 5 12 6 4 ( c ) and 5 12 ( d ) cages at 25, 100 and 260 K from MD simulation. Full size image In contrast to other clathrate hydrates, especially N 2 and O 2 hydrates, the structural behaviour of sI/sII CO hydrates has not been well established. For both sII N 2 and O 2 clathrates, the gas molecules in 5 12 6 4 cages are doubly occupied, shifted off the cage centre and oriented along the diagonals of their cubic unit cells [28] , [29] , while in 5 12 cages they are singly occupied at the cage centres and oriented along the <100> axes. MD simulations of the dynamic behaviour of N 2 and O 2 in sII clathrates indicate that the molecular positions and orientations are essentially the same for N 2 and O 2 and are independent of the cage size and distortion [30] . For comparison, the CO molecules in both 5 12 and 5 12 6 4 cages are off-centred. Notably, the CO molecules in 5 12 6 4 cages rotate around the centre by forming a cubic symmetry, and in 5 12 cages they are slightly off-centred with a pseudosphere configuration. In addition, an increased molecular freedom for CO molecules in large cages results in a distinct distribution of CO molecules with a hollow cubic geometry, whereas in small cages CO molecules are more confined/localized around the cage centre. With regard to the roles that dipole moment may play in the clathrate formation and stabilization, the present work does not provide a conclusive evidence. However, because CO has a small dipole moment, while N 2 is non-dipole (note they are isoelectronic), the different formation sequences observed for CO hydrates may presumably arise from the CO dipole effect during the nucleation stage, although the difference in the guest chemistry can also be a determining factor. More specifically, the dipole moment could act as a turbulence factor through the interaction with the dipolar water molecule during the nucleation stage. This is a process that is difficult to address experimentally and warrants future kinetic MD simulations using high-performance computing. For instance, the kinetic MD simulations may be performed by starting with a mixture of CO gas+water and determining the role of the dipole moment in the polyhedral cage formation at early stages of hydrate nucleation. Together with NMR or Raman/IR spectroscopic experiments, the formation sequence of sI and sII CO clathrates and associated crystallization and growth kinetics can be established. It should be stressed that the present work is relevant only to the growth of CO hydrates after their nucleation. The early nucleation of clathrate hydrates, as demonstrated by molecular simulations, typically involves densification and high local concentration of guest molecules to form individual cages [31] , [32] , [33] . These simulations also show that the clathrate nuclei are an amorphous mixture of polyhedral cages with structural motifs of a clathrate structure; hence, they do not have the same symmetry as the stable crystalline grains. In addition, the amorphous structure formed contains other types of cages that are not expected in an equilibrium hydrate structure. These characteristics of nucleation cannot be resolved using diffraction experiments. In summary, based on the time-dependent study of the clathrate hydrate formation in the CO-H 2 O system, we have demonstrated that sII hydrate can be formed in a time-evolving sequence after sI hydrate has initially crystallized. This finding validates previous hypotheses that sII CO hydrate would become more stable than sI CO hydrate when the concentration of CO molecules is saturated. This behaviour is associated with the difference in CO binding energy between 5 12 6 2 and 5 12 6 4 cages, where the 5 12 6 4 cage in the sII structure is energetically favoured over the 5 12 6 2 cage in the sI structure for double occupancy of CO molecules. More importantly, this is attributed to the crossover in the binding energy-cage occupancy space between the two cage types. As a result, a sII hydrate enclosing two CO molecules in 5 12 6 4 cages can be stabilized at certain P – T conditions through kinetically controlled cage filling. However, the (CO) 2 -(H 2 O) 28 clusters in an isolated state are energetically unfavourable and can readily dissociate into CO-(H 2 O) 28 and CO. Our MD simulations suggest that the interactions between adjacent cages including CO-H 2 O and CO-CO interactions provide a significant source of stability for the double-CO occupancy of hexakaidecahedral cage. Previous studies of CO hydrates indicate that both sI and sII CO hydrates may exist in the icy bodies of outer planets of the solar system, making them potentially important candidates for interpreting observed molecular anomalies [12] , [13] . Our comprehensive studies on their formation process, thermodynamic stability and encapsulation dynamics have provided valuable information for spectroscopic simulation and hence for detecting their occurrence in the solar system. Neutron diffraction data collection Time-of-flight neutron experiments were conducted at the HIPPO beamline, Los Alamos Neutron Science Center. The pressure cell was made of vanadium, which has a small coherent scattering for neutrons and can hold pressures up to 200 bar. To minimize the background of neutron patterns, deuterated water (D 2 O) instead of H 2 O was used for hydrate synthesis. Polycrystalline samples were prepared in a pressure vessel from ground D 2 O ice and gaseous CO at the initial pressure and temperature conditions (173 bar and 243 K) used in ref. 15 , 16 As confirmed by our neutron diffraction measurements, the sI CO clathrate was initially formed during the first 1–4 weeks at 173 bar and 243 K. A mixture of sI and sII CO clathrates was observed after 5 weeks, and, finally, a single-phase sII CO clathrate was obtained at ~100 bar and 252 K after 17 weeks ( Fig. 1 ). Rietveld refinement and MEM analysis All neutron diffraction data were analysed using the GSAS package [34] , and the CO positions in the clathrate cages were determined from the difference Fourier nuclear maps and refined by subsequent Rietveld analyses. The initial atomic coordinates for the D 2 O framework were taken from a previous neutron diffraction study of N 2 clathrate [29] . The D 2 O framework of sII CO clathrate and of the residual ice were both refined using Pauling’s half-hydrogen model with an average occupancy of 0.5 for each deuterium atom [35] . D 2 O in the framework can adopt six possible configurations as a result of the disordered orientation. However, diffraction experiments can only provide space- and time-averaged intra- and inter-molecular distances [29] , which may not reflect the instantaneous interactions between the framework cages and the guest molecules inside. The isotopic exchange between D in D 2 O ice and H atoms in atmospheric moisture was negligible and was ignored for all the refinements. To obtain the CO distributions in both small and large cages, difference nuclear Fourier maps were constructed after the best fit for the D 2 O framework was achieved. Our final Rietveld analysis revealed that in sII framework, each small cage is occupied by one CO molecule, whereas each large cage can be occupied by up to two CO molecules, resulting in a CO/D 2 O ratio of ~4/17 when all the cages are fully occupied. The refined occupancies for CO molecules indicated one molecule in the 5 12 cage and two in the 5 12 6 4 cage; they were fixed in the subsequent analysis to better constrain the CO distributions in cages. In this study, the distribution of CO molecules in sII hydrate over a range of temperatures was analysed by the MEM/Rietveld analyses using data from four detector banks at 2 θ =144.45°, 119.89°, 90.00° and 39.30°. The corresponding d -spacings are in the range of 0.5–10.5 Å ( Supplementary Fig. 5 ). The observed structure factors, F o , and standard uncertainties, (| F o |), were estimated with Alchemy [36] from relevant data in files output by GSAS and analysed by MEM with Dysnomia [37] . The unit cell was divided into 128 × 128 × 128 voxels. The detailed method for MEM analysis has been described in ref. 36 . DFT and MD calculations DFT was utilized in this work to provide further investigation on the stability of CO clathrate hydrates. The calculations utilized the Gaussian09 program package [38] . We optimized the structures of (H 2 O) 20 (5 12 cage in both sI and sII), (H 2 O) 28 (5 12 6 4 cage in sII) and (H 2 O) 24 (5 12 6 2 cage in sI and their corresponding CO complexes, at the level of Becke 3-Parameter for exchange and Lee, Yang and Parr parameters for correlation). DFT (B3LYP)/6-31+G(d) was used with the Coulomb-attenuating method [39] , [40] , [41] . All the stationary points were confirmed as minima by means of frequency calculations. To compare with our Rietveld refinement results of CO distributions in sII cages, we performed MD simulations with one CO molecule in each 5 12 cage and two CO molecules in 5 12 6 4 cage. A total of ~100,000 points from CO trajectories in 5 ns were projected on the a – b plane, and the cage centres of both 5 12 and 5 12 6 4 cages were set as the zero points. The MD calculations were carried out at temperatures ranging from 25 to 260 K in canonical NVT (N-moles, V-volume, and T-temperature) ensembles obtained using the Nosé–Hoover thermostat [42] , [43] . The dimensions of the simulation cells and their initial configurations were adopted using the experimental lattice parameters and geometries at corresponding temperatures. Three-dimensional periodic boundary conditions were applied. For the selection of proton configuration, the ‘ice rules’ (Bernal–Fowler ice rules) have been obeyed and the proton configuration with the minimum total dipole moment was selected. The TIP4P water model [44] was used to calculate the interaction between H 2 O molecules. The interactions between CO and H 2 O molecules were modelled by the summation of electrostatic and Lennard–Jones-type interactions. The parameters were taken from Manesh et al. [18] , who used them to study the distribution of CO molecules in sI clathrate. The bond length of the CO molecule was fixed at the experimental value, 1.128 Å (ref. 45 ). The Lennard–Jones parameters are 3.55 and 0.3089, kJ mol −1 for C atoms and 2.95 and 0.5120, kJ mol −1 for O atoms. The partial charges on the C and O atoms of the CO molecule were ±0.0223 in atomic units. The long-range electrostatic interactions were calculated with the Particle-Particle Particle-Mesh method [46] . The dimensions of the periodic simulation boxes were 34 × 34 × 34 3 , which were constructed by 2 × 2 × 2 unit cells. Therefore, the simulation domain included a total of 128 5 12 cages and 64 5 12 6 4 cages that incorporated a total of 1,088 water molecules. Each calculation was performed for 5.0 ns simulation time with a 1.0 fs time step. The RDF and spatial density distribution of CO molecules respective to the centre of the corresponding cages were obtained from MD trajectories. All MD simulations in this work were performed using the LAMMPS program suite [47] . How to cite this article: Zhu, J. et al. Encapsulation kinetics and dynamics of carbon monoxide in clathrate hydrate. Nat. Commun. 5:4128 doi: 10.1038/ncomms5128 (2014).